Photochemical activity of Titan’s low-altitude condensed haze Titan, the largest moon of Saturn and similar to Earth in many aspects, has unique orange-yellow colour that comes from its atmospheric haze, whose formation and dynamics are far from well understood. Present models assume that Titan’s tholin-like haze formation occurs high in atmosphere through gas-phase chemical reactions initiated by high-energy solar radiation. Here we address an important question: Is the lower atmosphere of Titan photochemically active or inert? We demonstrate that indeed tholin-like haze formation could occur on condensed aerosols throughout the atmospheric column of Titan. Detected in Titan’s atmosphere, dicyanoacetylene (C 4 N 2 ) is used in our laboratory simulations as a model system for other larger unsaturated condensing compounds. We show that C 4 N 2 ices undergo condensed-phase photopolymerization (tholin formation) at wavelengths as long as 355 nm pertinent to solar radiation reaching a large portion of Titan’s atmosphere, almost close to the surface. Titan, an orange-yellow coloured moon of Saturn, is unique in many ways. It is the second largest moon in our solar system and the only moon with a significant atmosphere—enriched with organics, in the atmosphere and on the surface. Unlike Earth, Titan’s atmosphere is oxygen-deficient, but instead dominated by nitrogen (>90%) and methane (~5%). Organics on Titan originate from photochemistry of N 2 and CH 4 in Titan’s upper atmosphere, initiated by solar wind particles and solar ultraviolet radiation. The earlier Voyager [1] and the current Cassini-Huygens [2] , [3] , [4] missions have provided tremendous insight into the atmosphere, aerosols and the surface—lakes, flows and dunes. The processes that control the observed Titan’s haze are still not well understood; in particular, at what altitudes the haze formation occurs. Pioneering laboratory studies showed that polymeric organic material, called tholins [5] , [6] , formed in discharge-driven reactions involving nitrogen, methane and other atmospheric compounds have optical properties similar to what had been deduced from observations of the Titan’s haze. Please note that ‘tholins’ are laboratory analogues of Titan’s haze particles, not the haze itself. Larger organics are currently thought to form high in Titan’s atmosphere at altitudes above 800 km ( [7] ), grow through coagulation in the lower atmosphere down to 500 km (refs 8 , 9 , 10 ), and finally rain down onto the surface. It has been suggested that ultraviolet-induced chemical processing (aging and hardening) of these aerosols can occur via solid-state polymerization [11] , [12] . Other observations and modelling studies infer that about 60% of the total column mass production of tholin-like aerosols may occur below 300 km (ref. 13 ) and that the production of large macromolecular particles peaks at ~100 km (ref. 14 ). This production includes condensation of simpler unsaturated organic compounds onto the larger haze particles at these cold low altitudes [15] . Below ~600 km, the gas composition and organic haze of Titan’s atmosphere significantly attenuate the greater part of high-energy electron, ion and photon radiation [16] . However, at longer wavelengths the solar spectrum is not significantly attenuated in Titan’s atmosphere until the 100 km altitude level is reached [17] . For example, ~99% of photons at wavelengths >220 nm make it through to lower altitudes [14] , [18] . The solar flux at 220 nm is estimated to be ~1 × 10 10 photons cm −2 nm −1 s −1 at 200 km, and at the same altitude the estimated solar flux at 350 nm is ~3 × 10 11 photons cm −2 nm −1 s −1 . The solar flux at 350 nm and at 200 km altitude is comparable to the upper atmosphere radiation field at shorter wavelengths that is important for inducing gas-phase upper atmospheric photochemistry. Even at lower altitudes (for example, at 70 km) the photon flux is not insignificant at both these wavelengths (~8 × 10 7 photons cm −2 nm −1 s −1 ). Thus, photochemical reactions that may occur in lower atmosphere (<600 km) involving longer wavelength solar photons (>200 nm) will have a significant role to play in Titan’s atmosphere and its photochemical evolution. Titan’s unusual dense and oxygen-depleted atmosphere has a wide variety of linear unsaturated polyynes—nitrogen-containing polycyanoacetylenes [19] , such as C 4 N 2 as well as polyacetylenes [20] and aromatic molecules [21] —that undergo photopolymerization forming complex tholin-like molecules, whose structure is still under intense investigation [22] . Recent laboratory studies showed that when these tholins come into contact with oxygen-bearing molecules such as water (surface/subsurface ice on Titan), result in the formation of complex prebiotic molecules such as amino acids [5] and nucleobases [23] , [24] . Thus, atmospheric aerosol photochemistry has a key role in the processes leading to the potential prebiotic chemistry on Titan’s surface [25] . As photoabsorption of condensed molecules can occur at longer wavelengths due to polarizability of condensed phase [26] exciton interactions [27] , [28] and spin-orbit coupling [29] , compared with their isolated molecular counterparts, the absorption of longer wavelength photons may trigger solid-state chemical processes with a sufficient yield to significantly affect low-altitude particle composition. Solid-state organic photochemistry could continue to altitudes as low as 50 km or below, leading to progressive conversion of Titan’s aerosols to complex polymeric organic material during the rain-down process. The three possible phases of organics in Titan’s atmosphere are schematically shown in Fig. 1 . Our laboratory studies presented here model the condensed small linear organic molecules that form a class of polyynes observed on Titan. While preparing a mixture of various possible polyynes and cyanopolyynes, as shown in Fig. 1 , would be a challenging task, the photochemical principles that govern these mixed monomers can be illustrated in the chemistry of one of these components alone, hence our choice to study single monomer condensates. Voyager 1 provided the first detection of crystalline organic ice in the Titan’s atmosphere—dicyanoacetylene (C 4 N 2 )—that confirmed the model expectation for gas condensation [30] , [31] , which prompted a series of laboratory work on C 4 N 2 in late 1990s (refs 32 , 33 ). Solid-state photopolymerization of these atmospheric ice condensates could be an important low-altitude source of macromolecular organic tholin-like material. The lower the altitude, the longer would be the wavelength of photons that could be causing photochemical activity in Titan’s atmosphere—all the way to the surface. Our laboratory simulations presented here show that photopolymerization of condensed unsaturated Titan’s volatiles indeed occurs at wavelengths at least as long as 355 nm. We conclude that contrary to the present understanding that Titan’s lower atmosphere is inert, our studies presented here show that Titan’s atmosphere is photochemically active even at lower altitudes and leads to the formation of complex tholin-like potential prebiotic molecules due to the penetrating longer wavelength photons. This is consistent with observations of Titan’s haze stretching between ~500 km and ~50 km above the surface [9] , containing several regions of haze (0, A, B and C) as recently characterized by the Cassini CIRS instrument [34] , [35] . 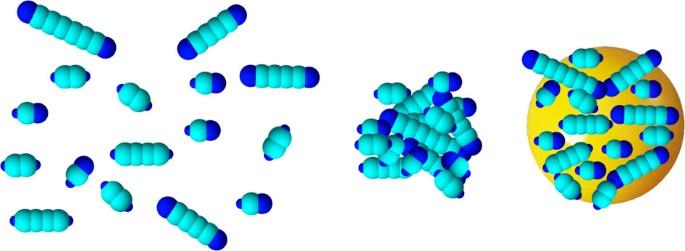Figure 1: Three phases of molecules in Titan’s atmosphere. Small molecules in Titan’s atmosphere could exist as isolated entities in the gas phase (left), condensed small molecules (middle) or accreted onto a larger aerosol particle (right). Gas-phase photochemistry is controlled by the molecular spectroscopic properties of the isolated molecules. In both condensed phases, additional photochemical pathways are triggered as detailed in the text. Figure 1: Three phases of molecules in Titan’s atmosphere. Small molecules in Titan’s atmosphere could exist as isolated entities in the gas phase (left), condensed small molecules (middle) or accreted onto a larger aerosol particle (right). Gas-phase photochemistry is controlled by the molecular spectroscopic properties of the isolated molecules. In both condensed phases, additional photochemical pathways are triggered as detailed in the text. Full size image Long-wavelength Titan aerosol analogue photochemistry We developed a laboratory study to investigate whether solid-state polymerization of large unsaturated organic molecules condensed on Titan’s aerosols could be induced by the photons (>220 nm) that still could penetrate through its atmosphere to low altitudes. For this simulation we chose C 4 N 2 given its known presence in Titan’s lower atmosphere [30] . Therefore, it also could serve as a model for other large condensed unsaturated organic compounds, particularly long linear chains of alternating single and multiple bonds, which are formed in this atmosphere. In the condensed phase, their interactions will be similar—whether between molecules with same molecular formula such as C 4 N 2 or a statistical distribution of a wide variety of molecules with varying chain lengths. As illustrated in Fig. 2 (top), the ultraviolet absorption spectrum of C 4 N 2 ice at 100 K has structure at <300 nm in agreement with the gas-phase spectrum [36] , [37] , [38] , [39] , but also a featureless long-wavelength absorption stretching to >360 nm, beyond where the gas-phase absorption ends. The broad continuum absorption at longer wavelengths than ~350 nm could be due to the weak singlet-triplet absorption amplified in the condensed phase, in agreement with detection of phosphorescence from the first triplet ( T 1 ) state of C 4 N 2 at ~390 nm (ref. 40 ). 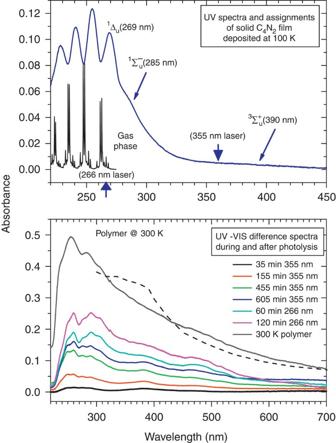Figure 2: Ultraviolet-visible spectra of dicyanoacetylene ice and its photoproduct tholin. Top: ultraviolet-visible absorption spectra of dicyanoacetylene (C4N2) solid films condensed at 100 K on a sapphire window. The gas-phase ultraviolet absorption spectrum of C4N2(39) is shown as black curve for comparison. Bottom: ultraviolet–visible absorption difference spectra obtained by subtracting the spectrum taken before laser photolysis from the spectra measured, first during photolysis at 355 nm, then followed by photolysis at 266 nm. Sample temperature was kept at 100 K during irradiation and then, subsequent to irradiation, warmed up to 300 K under vacuum (shifted curve on the top). The ultraviolet spectrum of the residual polymer (top curve) does not change significantly between 180 and 300 K, and it is similar to that of the conventional tholin (shown as dashed line) reported by Sagan and Khare6. Spikes and wiggles in the red curve at ~500 nm are artefacts from the ultraviolet lamp profile. Figure 2: Ultraviolet-visible spectra of dicyanoacetylene ice and its photoproduct tholin. Top: ultraviolet-visible absorption spectra of dicyanoacetylene (C 4 N 2 ) solid films condensed at 100 K on a sapphire window. The gas-phase ultraviolet absorption spectrum of C 4 N 2 ( [39] ) is shown as black curve for comparison. Bottom: ultraviolet–visible absorption difference spectra obtained by subtracting the spectrum taken before laser photolysis from the spectra measured, first during photolysis at 355 nm, then followed by photolysis at 266 nm. Sample temperature was kept at 100 K during irradiation and then, subsequent to irradiation, warmed up to 300 K under vacuum (shifted curve on the top). The ultraviolet spectrum of the residual polymer (top curve) does not change significantly between 180 and 300 K, and it is similar to that of the conventional tholin (shown as dashed line) reported by Sagan and Khare [6] . Spikes and wiggles in the red curve at ~500 nm are artefacts from the ultraviolet lamp profile. Full size image Details of the laboratory simulation apparatus are summarized in Methods and further details are available in the Supplementary Material for this article. Laser photolysis experiments at the Jet Propulsion Laboratory were conducted at three wavelengths: 532, 355 and 266 nm, which were obtained by second, third and fourth harmonic generation of a 5-ns pulsed Nd-YAG. Photon fluxes used in these experiments were typically ~1 × 10 17 , ~3 × 10 16 and ~5 × 10 16 photons cm −2 s −1 at 532, 355 and 266 nm, respectively. To avoid multiphoton processes, the initial laser beam of ~3 mm diameter was expanded to ~20 mm using a 10-cm focal-length quartz lens. The experiments were designed to conserve the C 4 N 2 that was difficult to synthesize. The C 4 N 2 ice sample was first irradiated with the 532 nm laser for several hours at ~0.15 W cm −2 flux. No detectable change in the infrared spectra (2,244 cm −1 ) was observed from the photolysis at this wavelength. The same C 4 N 2 ice was then subjected to 355 nm irradiation, which resulted in depletion of ~7% of the infrared absorption over 8 h of irradiation. As the degree of processing due to 355 nm irradiation was small, the same sample was then exposed to the 266 nm laser beam, which resulted in significantly more (a total of ~50%) depletion of the infrared absorption. In subsequent experiments, the 532 nm irradiation was omitted. We are confident that, although laser-desorption as a competing process could not be completely ruled out, it is not the dominant process. If it were, one should observe only a decrease in the monomer band and not an increase in the broad absorption that persists even after sublimation of the monomer C 4 N 2 . We also conducted several control experiments where the C 4 N 2 ices were (a) not irradiated, (b) only irradiated with 355 nm laser, and (c) only irradiated with 266 nm laser. Unirradiated C 4 N 2 films did not yield a residue on warm-up. Irradiation only with 266 nm laser resulted in similar photopolymerization process as with 355 nm irradiation before the 266 nm irradiation. In both 266 nm laser and mercury (Hg) lamp photolysis experiments, the latter carried out at the University of Provence, France, the photopolymer remaining at room temperature under vacuum was similar—an orange-brown non-volatile film. A photograph of the experimental photopolymerized aerosol analogue made at the Jet Propulsion Laboratory is shown in Fig. 3 . The structured vibronic absorption of condensed C 4 N 2 ice in the ultraviolet (200–300 nm) decreases during 355 nm irradiation due to photopolymerization, whereas the broad and structure-less absorption increases, indicating photoproduct absorption/scattering to be stronger than the monomer C 4 N 2 absorption in the ultraviolet. This trend continues with 266 nm laser photolysis ( Fig. 2 , bottom). Differencing spectra taken before and after the initiation of irradiation at each wavelength reveals the extent of sample processing. As shown in Fig. 4 (top), photolysis at 355 nm results in depletion of the 2,244 cm −1 band and an increase of a broader absorption around the depleted peak, also due to CN stretching of the polymer ( Fig. 4 , top inset). Irradiation at 266 nm resulted in a significant decrease of monomer absorption at 2,244 cm −1 , but the increase in the broad absorption was not relatively as significant as in the 355 nm photolysis ( Fig. 4 , middle). 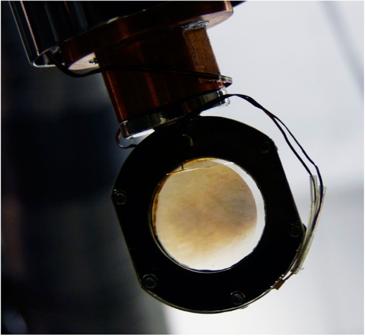Figure 3: Photochemically produced tholin under simulated Titan’s lower atmospheric conditions. Photograph of the non-volatile polymeric residue film remaining on the sapphire substrate window after warmup to 300 K under vacuum. This residue was formed during the laser photolysis of condensed C4N2molecules at 266 nm at the Jet Propulsion Laboratory (JPL). Similar orange-brown tholin-like non-volatile polymeric residues were observed during several similar experiments at JPL and the University of Provence, France. Figure 3: Photochemically produced tholin under simulated Titan’s lower atmospheric conditions. Photograph of the non-volatile polymeric residue film remaining on the sapphire substrate window after warmup to 300 K under vacuum. This residue was formed during the laser photolysis of condensed C 4 N 2 molecules at 266 nm at the Jet Propulsion Laboratory (JPL). Similar orange-brown tholin-like non-volatile polymeric residues were observed during several similar experiments at JPL and the University of Provence, France. 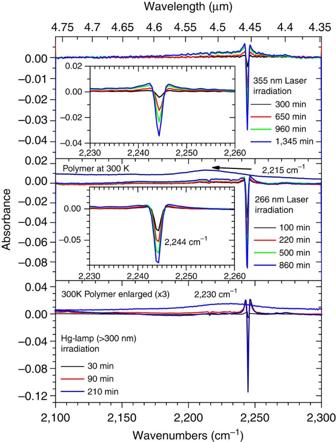Figure 4: Infrared spectra of dicyanoacetylene ice and their changes during laser photolysis. Results of the laser irradiation experiments conducted at the Jet Propulsion Laboratory (top and middle) and Hg-lamp irradiation experiments conducted at the University of Provence, France (bottom). The polymer residual spectra (middle and bottom boxes) were referenced to background spectra taken before C4N2was deposited, whereas all the other spectra show differences between the spectra after irradiation at the specified wavelength and duration and the spectra before irradiation. Negative absorbance means depletion of the spectral feature. Positive absorbance is due to the appearance of a new spectral feature. Top: laser photolysis at 355 nm. Depletion of the absorption at 2,244 cm−1and increase in polymer/intermediate photoproducts absorption (broad 2,235–2,250 cm−1) can clearly be seen. Middle: laser photolysis at 266 nm resulting in more significant depletion. Broad 2,215 cm−1CN stretching band, measured at 300 K after warm-up, is the infrared spectrum for the orange-brown coloured non-volatile polymer (Fig. 3). Bottom: high-pressure Hg-lamp photolysis (photons <300 nm filtered out) showing spectra similar to 355 nm laser photolysis (top panel). Full size image Figure 4: Infrared spectra of dicyanoacetylene ice and their changes during laser photolysis. Results of the laser irradiation experiments conducted at the Jet Propulsion Laboratory (top and middle) and Hg-lamp irradiation experiments conducted at the University of Provence, France (bottom). The polymer residual spectra (middle and bottom boxes) were referenced to background spectra taken before C 4 N 2 was deposited, whereas all the other spectra show differences between the spectra after irradiation at the specified wavelength and duration and the spectra before irradiation. Negative absorbance means depletion of the spectral feature. Positive absorbance is due to the appearance of a new spectral feature. Top: laser photolysis at 355 nm. Depletion of the absorption at 2,244 cm −1 and increase in polymer/intermediate photoproducts absorption (broad 2,235–2,250 cm −1 ) can clearly be seen. Middle: laser photolysis at 266 nm resulting in more significant depletion. Broad 2,215 cm −1 CN stretching band, measured at 300 K after warm-up, is the infrared spectrum for the orange-brown coloured non-volatile polymer ( Fig. 3 ). Bottom: high-pressure Hg-lamp photolysis (photons <300 nm filtered out) showing spectra similar to 355 nm laser photolysis (top panel). Full size image Nature of the photopolymer During warm-up under vacuum, spectral features of non-volatile photopolymer emerge in the ultraviolet and infrared spectra at temperatures beyond the sublimation temperature of C 4 N 2 (~160 K) to room temperature. The polymer should be forming even at 100 K during photolysis or between 100 and 160 K during the warm-up, but its spectral signatures, as they are broad, are obscured by monomer spectra before the monomer sublimes at ~160 K ( Supplementary Fig. S1 ). For purposes of confirmation, we performed a similar C 4 N 2 ice irradiation at the University of Provence (Marseille, France), using a conventional high-pressure Hg-lamp equipped with a <300 nm cutoff filter. The results obtained were very similar to the 355 nm laser irradiation experiments, as can be seen from the infrared spectra shown in Fig. 4 (bottom). The differences in the polymer absorption maximum when irradiated with the 266 nm laser (2,215 cm −1 ) or with the Hg lamp at >300 nm (2,230 cm −1 ), shown in Fig. 4 , could be due to the difference in reaction pathways accessible for photons below 280 nm versus above 300 nm. The structure-less ultraviolet spectrum resembles more closely the tholin ultraviolet-visible spectra reported by Sagan and Khare [6] , shown as dashed curve in Fig. 2 , than the spectra of Imanaka et al . [41] On the other hand, Fourier transform infrared (FTIR) spectra in the 4,000–1,600 cm −1 region are similar ( Fig. 5 ) to the infrared spectra of discharge-generated polymer reported by Imanaka et al . [41] , [42] In spite of the difference in preparation methods (gas-phase discharge at various pressures versus condensed-phase photochemistry) and the initial conditions (N 2 +CH 4 versus C 4 N 2 ), these qualitative similarities in the optical properties of the non-volatile polymer (tholin) reveal that these materials have very similar chemical structures. The actual structural properties of tholins are not known and are expected to be diverse, both at the molecular structure (chemical bonding) level and at the supramolecular structure (three-dimensional polymer structures) level. We prefer not to over interpret these data, but to show that tholins—though could have similar spectral properties may have diverse molecular and supramolecular aerosol structures. 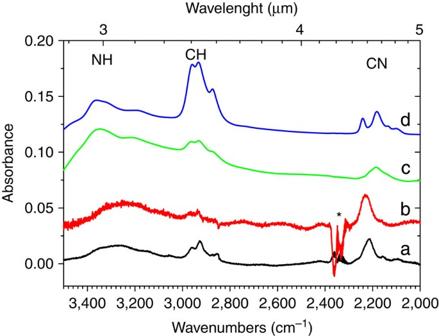Figure 5: A comparison of the infrared spectra of tholins synthesized in the gas and condensed phases. Infrared spectra of tholin-like photopolymers at room temperature compared with tholins made from conventional discharge experiments by Imanaka41,42. Method of preparation of tholin, bottom to top (a–d): JPL 266 nm laser photolysis (a); Marseille Hg lamp (>300 nm) pholysis (b); 10% methane in nitrogen discharge41at 26 Pa (c) and at 160 Pa (d). An excellent comparison between longer wavelength photochemical polymer spectra (JPL: 266 nm; Marseille >300 nm) and with the discharge-made tholins spectra can be seen. In our spectra the ratio of CN to CH and NH, band strengths is different (more CN) compared to Imanaka’s data, because in our experiments far-less hydrogen is available (either as traces of H2O impurity, or intentionally added H2O or other hydrocarbons such as CH4or C2H2). *Gas-phase CO2residual absorption. Figure 5: A comparison of the infrared spectra of tholins synthesized in the gas and condensed phases. Infrared spectra of tholin-like photopolymers at room temperature compared with tholins made from conventional discharge experiments by Imanaka [41] , [42] . Method of preparation of tholin, bottom to top ( a – d ): JPL 266 nm laser photolysis ( a ); Marseille Hg lamp (>300 nm) pholysis ( b ); 10% methane in nitrogen discharge [41] at 26 Pa ( c ) and at 160 Pa ( d ). An excellent comparison between longer wavelength photochemical polymer spectra (JPL: 266 nm; Marseille >300 nm) and with the discharge-made tholins spectra can be seen. In our spectra the ratio of CN to CH and NH, band strengths is different (more CN) compared to Imanaka’s data, because in our experiments far-less hydrogen is available (either as traces of H 2 O impurity, or intentionally added H 2 O or other hydrocarbons such as CH 4 or C 2 H 2 ). *Gas-phase CO 2 residual absorption. Full size image In the condensed phase, in addition to normal spin-allowed ultraviolet absorption, photochemical reactions can also occur through absorption of light at longer wavelengths directly into the triplet-excited states, which have strong radical character. In the case of C 4 N 2 , the spin-allowed ultraviolet absorption occurs at <300 nm and spin-forbidden absorption occurs at >300 nm—hence very efficient photodepletion of monomer at 266 nm compared to irradiation at 355 nm ( Fig. 2 ). Larger unsaturated organics condensed onto aerosols likely have both spin-allowed strong and spin-forbidden (condensed-phase enhanced) weak photoabsorptions and similar solid-state photoprocessing potential. It is known that gas-phase C 4 N 2 could dissociate with 248 nm light [43] , [44] resulting in the formation of CN and the CCCN radicals. Hence, the 266 nm photochemistry is likely to be controlled by dissociation products. Results discussed above indicate that singlet-triplet absorption-driven (355 nm irradiation) photochemical processes involves triplet C 4 N 2 molecules reacting with other C 4 N 2 molecules in its surrounding, resulting in the formation of the photopolymer ( Fig. 6 ), whose CN stretching vibrational absorption remains around 2,244 cm −1 , but is much broader. Upon warm-up this band shifts to 2,225 cm −1 , once the monomer is sublimed above 160 K. On the other hand, singlet-excitation-driven (<280 nm) photochemical processes result in molecular dissociation of C 4 N 2 into C 3 N and CN radicals as well as photopolymerization ( Fig. 6 ). The dissociation products recombine and react with other molecules during the warm-up until the monomer C 4 N 2 sublimes, at which time the polymer absorption ~2,215 cm −1 can clearly be seen. These mechanisms, qualitatively highlighted in Fig. 6 , would be applicable to mixed cyanopolyynes and polyynes, known to be present in Titan’s atmosphere. Both ultraviolet and infrared spectra of the polymer do not change significantly between 180 and 300 K, once the volatile monomer has evaporated above 160 K. Slight shifts in the broad absorption maxima of the polymer in 266 nm laser, 355 nm laser and >300 nm Hg-lamp studies, 2,215 cm −1 , 2,225 cm −1 , 2,230 cm −1 , respectively, could be due to different local environments around the –CN functional group of the photopolymer. It is known that the CN stretching frequency shifts based on the structural environment around it—less or more polar and less or more hydrogen bonding [45] . 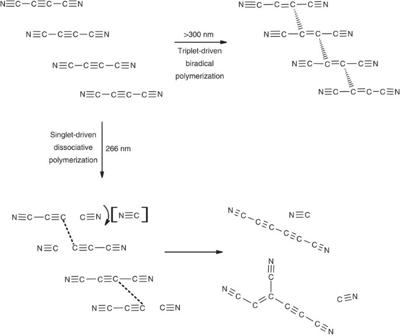Figure 6: Possible reaction pathways for longer wavelength production of tholins in condensed phase. Proposed mechanisms for the longer wavelength (ultraviolet-visible photons) triplet excitation-driven and shorter wavelength (ultraviolet photons) singlet-excitation-driven photopolymerization of C4N2in the condensed aerosol phase. Broken lines are not bonds, but represent new bond formation in progress. Radical centers are not specifically shown to avoid congestion in structures. While longer wavelengths result in more uniform polymerization, shorter wavelengths result in dissociation of parent C4N2to C3N and CN radicals that react to form a wide distribution of polymers. In both cases, monomer molecules accreted on an existing aerosol particle (Fig. 1) could chemically bind to this haze particle, increasing its size and modifying it chemically on its surface—a process that could be critical to Titan’s atmospheric chemistry, but not considered previously. Figure 6: Possible reaction pathways for longer wavelength production of tholins in condensed phase. Proposed mechanisms for the longer wavelength (ultraviolet-visible photons) triplet excitation-driven and shorter wavelength (ultraviolet photons) singlet-excitation-driven photopolymerization of C 4 N 2 in the condensed aerosol phase. Broken lines are not bonds, but represent new bond formation in progress. Radical centers are not specifically shown to avoid congestion in structures. While longer wavelengths result in more uniform polymerization, shorter wavelengths result in dissociation of parent C 4 N 2 to C 3 N and CN radicals that react to form a wide distribution of polymers. In both cases, monomer molecules accreted on an existing aerosol particle ( Fig. 1 ) could chemically bind to this haze particle, increasing its size and modifying it chemically on its surface—a process that could be critical to Titan’s atmospheric chemistry, but not considered previously. Full size image In our studies presented here, during the photolysis and warm-up, additional reactions with traces of H 2 O impurity, or intentionally added H 2 O, or other hydrocarbons such as CH 4 or C 2 H 2 , result in the formation of CH and NH functional groups into the polymer, whose spectra at room temperature are very similar to the tholin infrared spectra made from conventional discharge experiments [41] ( Fig. 5 ). Based on this observation, we conclude that the intermediate photoproducts are very reactive towards hydrogen-containing molecules. Though water is sparse, hydrocarbons are abundant on Titan and similar photochemical processes are expected to occur in the Titan’s atmosphere. In addition, we investigated the efficiency of photoprocessing by monitoring the time evolution of the C 4 N 2 infrared absorption on irradiation at 355 and 266 nm. 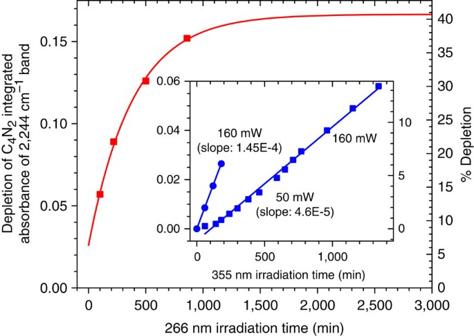Figure 7: Photodepletion kinetics of dicyanoacetylene ice. Time variation of change in absorption at 2,244 cm−1when C4N2film at 100 K is photolysed at 355 nm (inset) and 266 nm. As expected for a forbidden and weak singlet-triplet absorption-induced photochemistry, the depletion of C4N2is linearly proportion to the irradiation time when exposed at 355 nm, representing initial stages of an exponential process. Only 14% of C4N2was depleted after ~1,400 min irradiation at ~50 mW cm−2. The last three points on the lower curve (filled squares) were obtained using higher laser power (160 mW cm−2or 8 mJ per pulse), whereas the rest of the data were derived using a 50 mW cm−2(2.5 mJ per pulse) laser power. Linearity of this curve when fluence is converted to time clearly indicates that the 355 nm photochemistry is a one-photon process. We also plotted these three points with 160 mW cm−2laser power separately (filled circles). As discussed in the text, the slopes of these two curves scale linearly with the laser fluencies—confirming that the 355 nm photochemistry is indeed a one-photon process. The 266 nm photolysis through singlet-singlet excitation follows a monoexponential curve with over 35% depletion within the first 800 min of irradiation at 120 mW cm−2. Extrapolation towards the longer durations of the 266 nm photolysis may not be accurate due to simultaneous increase in extinction of the film at this wavelength from the formation of new products. Figure 7 shows the change in C 4 N 2 infrared absorption with exposure time. The change during 355 nm irradiation is linear with photon flux (dose), indicating that the photochemistry is due to weak electronic transitions (singlet-triplet), falling in a small linear segment of a first-order reaction (only ~13% depletion in ~1,300 min) that would have developed into a nonlinear exponential behaviour on prolonged photolysis. Continuing with the photolysis at 266 nm resulted in more rapid depletion of C 4 N 2 , following a single exponential behaviour, in accordance with first-order exponential process [46] (a total of ~48% depletion after 860 min irradiation at 266 nm). Figure 7: Photodepletion kinetics of dicyanoacetylene ice. Time variation of change in absorption at 2,244 cm −1 when C 4 N 2 film at 100 K is photolysed at 355 nm (inset) and 266 nm. As expected for a forbidden and weak singlet-triplet absorption-induced photochemistry, the depletion of C 4 N 2 is linearly proportion to the irradiation time when exposed at 355 nm, representing initial stages of an exponential process. Only 14% of C 4 N 2 was depleted after ~1,400 min irradiation at ~50 mW cm −2 . The last three points on the lower curve (filled squares) were obtained using higher laser power (160 mW cm −2 or 8 mJ per pulse), whereas the rest of the data were derived using a 50 mW cm −2 (2.5 mJ per pulse) laser power. Linearity of this curve when fluence is converted to time clearly indicates that the 355 nm photochemistry is a one-photon process. We also plotted these three points with 160 mW cm −2 laser power separately (filled circles). As discussed in the text, the slopes of these two curves scale linearly with the laser fluencies—confirming that the 355 nm photochemistry is indeed a one-photon process. The 266 nm photolysis through singlet-singlet excitation follows a monoexponential curve with over 35% depletion within the first 800 min of irradiation at 120 mW cm −2 . Extrapolation towards the longer durations of the 266 nm photolysis may not be accurate due to simultaneous increase in extinction of the film at this wavelength from the formation of new products. Full size image We also conducted experiments to rule out the possibility whether multiphoton processes could have resulted in the observed photochemistry. The experiments conducted in France were conducted using a 150 W high-pressure Mercury lamp that was flooded (without focusing) on the sample after cutting out the shorter wavelengths below 300 nm using a glass filter. These results are very similar to the results from defocused laser irradiation. Further, we changed the pulse energy ( E L ) of 355 nm laser by a factor of 3 (from 50 to 160 mW cm −2 before defocusing the laser), keeping the repetition rate at 20 Hz. The photolysis yields (φ) plotted in the insert of Fig. 7 (after converting normalizing photon flux to time) fall linearly on the curve at the last three-irradiation points. Also plotted in Fig. 7 are the photolysis yields for 160 mW cm −2 irradiation (the last four points on the main curve). The slopes of these two curves give the photolysis yields per minute at these two laser fluencies. While a single-photon process follows the equation (φ)= k × E L ; a two-photon process obeys a quadratic dependence (φ)= k ′ × ( E L ) 2 . Ratios of photolysis yields at two laser fluencies E L1 and E L2 should follow (φ 1 /φ 2 )=( E L1 / E L2 ) for single-photon process and ( E L1 / E L2 ) 2 for a two-photon process. The laser fluence ratio (160 mW/50 mW) is 3.2 for single-photon and 10.24 for two-photon processes. The observed photolysis yield ratio (φ 1 /φ 2 ) of 3.15 ( Fig. 7 ) clearly demonstrates that the photoabsorption and the photochemistry with 355 nm laser irradiation presented here are linear one-photon processes, not involving nonlinear multiphoton processes. Laser irradiation at 266 nm is done under similar conditions (~0.12 W cm −2 before defocusing) and we infer a single-photon-induced photochemical process at this wavelength as well. Under our experimental conditions (~10 −9 mbar vacuum) C 4 N 2 starts to sublime around 160 K. No sign of sublimation is detected at 100 K. Based on these observations, for similar monomer molecules, we expect the sticking coefficient in Titan’s atmosphere at much higher pressures and similar temperatures to be close to unity. Experimental data presented here demonstrate that solar radiation at wavelengths that penetrate deep into Titan’s atmosphere, down to 200 km and below, can initiate a new source of tholin-like haze production from the condensates in this altitude range. As the sedimentation velocity in this region is very slow, of order ~0.03 cm s −1 at ~100 km altitude [22] , aerosol particles stay within the haze layer for ~10 Earth years or ~3 × 10 8 s. Solar photon flux at 10 AU is ~14 W m −2 and photons between 200 and 350 nm constitute ~5% of the total energy flux, resulting in ~0.7 or 7 × 10 −5 W cm −2 or ~10 14 photons cm −2 s −1 (over 200–350 nm) or ~6 × 10 11 photons cm −2 s −1 nm −1 . The laboratory dose was typically 0.15 W cm −2 , which amounts to ~2,000 times more flux than received by Titan’s atmosphere at these wavelengths. As seen in Fig. 7 , photochemical polymerization at 355 nm of a condensed C 4 N 2 film (~200 nm thick) is ~13% over 1,340 min (84,000 s) and 0.05 W cm −2 flux, which corresponds to ~6 × 10 7 s on Titan, which is a factor of 5 less time that an aerosol particle spends in Titan’s atmosphere. So significant photopolymerization processing in Titan’s atmosphere is possible from weakly allowed spin-forbidden photoexcitations, resulting in solid-state radical reactions. On the other hand, photopolymerization due to 266 nm photons, caused by strongly allowed photoexcitation, occurs much faster, ~35% yield over 860 min (21,600 s) at 0.12 W cm −2 , which corresponds to ~4 × 10 7 s on Titan, an order of magnitude less than the residence time of aerosols in Titan’s condensed haze layer. Based on these data we infer that significant photochemical polymerization is expected to occur involving spin-allowed strong ultraviolet absorption by Titan’s aerosol molecules. Chemical models predict the formation of unsaturated organic molecules even larger than C 4 N 2 in Titan’s atmosphere [47] . As with C 4 N 2 , the larger molecules will condense into ices in the lower atmosphere. The gas-phase spectra of such molecules will have absorption longward of the C 4 N 2 gas-phase absorption, and in condensed phase these absorption spectra would be shifted to even longer wavelengths. Therefore, solar radiation out to visible wavelengths penetrating to Titan’s lower atmosphere may initiate production of photopolymerization of condensed organic aerosols not previously accounted for and can provide a mechanism for the majority of tholin formation predicted to occur at low altitudes. We conclude that Titan’s lower atmosphere is more photochemically active than so far assumed. In addition, experimental results presented here can be extrapolated to shorter wavelength solar radiation at higher altitudes, exposure to which should lead to condensed-phase processing of accumulations of unsaturated organic molecules as previously suggested [11] , [12] . Thus, tholin-like haze formation occurs by a variety of different photo-initiated processes throughout the whole atmospheric column of Titan. Titan organic aerosol synthesis and photochemistry experiment Dicyanoacetylene (C 4 N 2 ) was synthesized according to a well-established procedure reported in the literature [48] , [49] . These molecules are highly unstable and hazardous. Hence we developed a synthesis laboratory adjacent to the spectroscopy and photochemistry lab. C 4 N 2 was prepared and used immediately to make ice films at 100 K. During the vapour deposition of C 4 N 2 on the cryogenic window (Sapphire or KBr, both transmit ultraviolet and infrared for the CN stretch around 2,244 cm −1 , sapphire cutoff is ~1,600 cm −1 , whereas KBr is transparent down to 450 cm −1 ), the sample window was kept at 100 K. Bulk C 4 N 2 was kept at around −30 °C during the sublimation into the ice chamber and subsequently after the preparation of ice films, the C 4 N 2 container was removed from the vacuum line and was stored in an −80 °C ice chest or in a dry-ice container. Details of the experimental system are shown in Supplementary Figs S2 and S3 . The experimental system in which thin films of C 4 N 2 ices were generated consisted of a closed-cycle helium cryostat (Advanced Research Systems) that cooled the substrate window (Sapphire or KBr). C 4 N 2 was deposited from gas phase onto the window cooled to 100 K, a temperature relevant to Titan’s lower atmosphere. All the irradiation experiments were done at 100 K, and at the end of the experiments temperature was raised at 5 K min −1 to room temperature. Infrared spectra were collected during the entire warm-up. Optical configuration of the substrate, FTIR, fibre optics ultraviolet-visible spectrometers and irradiation lasers were such that sample was not moved during simulataneous ultraviolet and infrared spectral measurements or during laser irradiation ( Supplementary Fig. S3 ). Growth of C 4 N 2 films were controlled such that the 2,244 cm −1 infrared absorption band reached an absorbance of ~0.1. This process ensured that enough material was deposited to allow measurable photoprocessing, but not too much material that would result in nonlinear absorption properties (>1.0 Abs) or scattering. Both the laser beam and the infrared beam from the FTIR spectrometer illuminated the whole ~20 mm sapphire window and the C 4 N 2 film, while ultraviolet-visible spectra were collected from a ~5 mm diameter area in the centre of the window. To avoid inducing additional photoprocessing due to ultraviolet light that may interfere with the kinetic analysis, we did not monitor the sample evolution using ultraviolet spectra, but instead used the mid-infrared band at 2,244 cm −1 . We used the sapphire window for its excellent optical quality in the ultraviolet-visible spectral region (>180 nm) all the way into the mid-infrared (>1,600 cm −1 ), enabling simultaneous ultraviolet and infrared spectroscopy. In few experiments we used KBr substrate, gaining access to the infrared (>500 cm −1 ) at the cost of ultraviolet spectra. In these studies, other strong infrared bands of C 4 N 2 (738 and 1,160 cm −1 ) with relative peak heights of ~10% compared with the 2,244 cm −1 band, as well as a number of very weak combination bands between 2,250 and 3,400 cm −1 were observed ( Supplementary Fig. S4 ), in accordance with earlier studies of C 4 N 2 in Ar matrices [50] . For this reason, we used the strongest 2,244 cm −1 CN asymmetric stretch band for quantitative data analysis. Ultraviolet and FTIR spectra were measured on C 4 N 2 ice at 100 K simultaneously on the same sample around the same time, enabling a good comparison between the ultraviolet and infrared spectra. While increasing scattering was observed with increasing ice thickness in the FTIR spectra, ultraviolet spectra were a convolution of electronic absorption and interference due to reflections caused by the C 4 N 2 ice film on the sapphire window. These interference modulations were used to derive film thickness assuming a refractive index of 1.45, typical of many refractory organics such as polycyclic aromatic hydrocarbons (PAHs). Laser and lamp photochemistry A Nd-YAG laser (Quantel Brio) with second, third and fourth harmonic generation at 532, 355 and 266 nm was used for photochemistry. Laser light was defocused as explained below to avoid multiphoton processes such as resonance-enhanced multiphoton ionization or two-photon excitation into electronically excited states. Under solar radiation conditions such multiphoton absorption processes are negligible and in the laboratory these processes must be avoided to have a valid Titan simulation. The diameter of laser light was initially ~5 mm. A 10 cm focal length quartz biconvex lens was placed at ~50 cm from the cryostat to result in a beam diameter of ~20 mm on the optical window containing C 4 N 2 sample. Photon fluxes used in these experiments were typically ~1 × 10 17 , ~3 × 10 16 and ~5 × 10 16 photons cm −2 s −1 at 532, 355 and 266 nm, respectively, before defocusing. A ultraviolet-visible absorption spectrograph (Ocean Optics USB4000) was used to detect optical changes between 200 and 1,000 nm, a FTIR spectrometer (Thermo Nicolet 6700) covering 1 micron to 20 microns (10,000 to 500 cm −1 ), sapphire substrate cutoff ~1,600 cm −1 . Though the substrate window could be rotated around 360° in the vacuum chamber, to enhance the accuracy of spectral changes, the organic film substrate window was kept in the same position during the entire experiment (after initial deposition) enabling simultaneous laser irradiation, ultraviolet and infrared spectral measurements. How to cite this article: Gudipati, M. S. et al . Photochemical activity of Titan’s low-altitude condensed haze. Nat. Commun. 4:1648 doi: 10.1038/ncomms2649 (2013).